High-throughput imaging of self-luminous objects through a single optical fibre Imaging through a single optical fibre offers attractive possibilities in many applications such as micro-endoscopy or remote sensing. However, the direct transmission of an image through an optical fibre is difficult because spatial information is scrambled upon propagation. We demonstrate an image transmission strategy where spatial information is first converted to spectral information. Our strategy is based on a principle of spread-spectrum encoding, borrowed from wireless communications, wherein object pixels are converted into distinct spectral codes that span the full bandwidth of the object spectrum. Image recovery is performed by numerical inversion of the detected spectrum at the fibre output. We provide a simple demonstration of spread-spectrum encoding using Fabry–Perot etalons. Our technique enables the two-dimensional imaging of self-luminous (that is, incoherent) objects with high throughput in principle independent of pixel number. Moreover, it is insensitive to fibre bending, contains no moving parts and opens the possibility of extreme miniaturization. Optical imaging devices have become ubiquitous in our society, and a trend toward their miniaturization has been inexorable. In addition to facilitating portability, miniaturization can enable imaging of targets that are difficult to access. For example, in the biomedical field, miniaturized endoscopes can provide microscopic images of subsurface structures within tissue [1] . Such imaging is generally based on the use of miniaturized lenses, though for extreme miniaturization, lensless strategies may be required [2] . Particularly attractive is the possibility of imaging through a single, bare optical fibre. The transmission of spatial information through an optical fibre can be achieved in many ways [3] , [4] . One example is by modal multiplexing where different spatial distributions of light are coupled to different spatial modes of a multimode fibre. Propagation through the fibre scrambles these modes, but these can be unscrambled if the transmission matrix [5] , [6] of the fibre is measured a priori [7] , [8] , [9] , [10] , [11] , [12] . Such spatio-spatial encoding can lead to high information capacity [13] , but suffers from the problem that the transmission matrix is not robust. Any motion or bending of the fibre requires a full recalibration of this matrix [10] , [11] , which is problematic while imaging. A promising alternative is spatio-spectral encoding, since the spectrum of light propagating through a fibre is relatively insensitive to fibre motion or bending. Moreover, such encoding presumes that the light incident on the fibre is spectrally diverse, or broadband, which is fully compatible with our goal here of imaging self-luminous sources. Techniques already exist to convert spatial information into spectral information. For example, a prism or grating maps different directions of light rays into different colours. By placing a miniature grating and lens in front of an optical fibre, directional (spatial) information can be converted into colour (spectral) information, and launched into the fibre. Such a technique has been used to perform one-dimensional (1D) imaging of transmitting or reflecting [4] , [14] , [15] , [16] or even self-luminous [17] , [18] objects, where two-dimensional (2D) imaging is then obtained by a mechanism of physical scanning along the orthogonal axis. Alternatively, scanningless 2D imaging with no moving parts has been performed by angle–wavelength encoding [4] or fully spectral encoding using a combination of gratings [19] or a grating and a virtual image phased array [20] , [21] . These 2D techniques have only been applied to non-self-luminous objects. Such techniques of spectral encoding using a grating have been implemented in clinical endoscope configurations only recently. To our knowledge, the smallest diameter of such an endoscope is 350 μm, partly limited by the requirement of a miniature lens in the endoscope [22] . A property of prisms or gratings is that they spread different colours into different directions. For example, in the case of spectrally encoded endoscopy [16] , broadband light from a fibre is collimated by a lens and then spread by a grating into many rays travelling in different directions. Such a spreading of directions defines the field of view of the endoscope. If we consider the inverse problem of detecting broadband light from a self-luminous source using the same grating/lens configuration, we find that because of this property of directional spreading, only a fraction of the spectral power from the source is channelled by the grating into the fibre. The rest of the power physically misses the fibre entrance, which plays the role of a spectral slit, and gets lost. Indeed, if the field of view is divided into M resolvable directions (object pixels), then at best only the fraction 1/ M of the power from each pixel can be detected. Such a scaling law is inefficient and prevents the scaling of this spectral encoding mechanism to many pixels (a similar problem occurs when using a randomly scattering medium instead of a grating [23] , [24] ). Given that the power from self-luminous sources is generally limited, it certainly is desirable to not throw away most of this power. Our solution to this problem involves the use of a spectral encoder that does not spread the direction of an incoming ray, imprints a code onto the ray spectrum depending on the ray direction, and this code occupies the full bandwidth of the spectrum. As a result of these properties, the fraction of power that can be detected from any given object pixel is roughly fixed and does not decrease as 1/ M . We call our encoder a spread-spectrum encoder (SSE). Indeed, there is a close analogy with strategies used in wireless communication [25] . While the spectral encoding techniques described above that involve gratings perform the equivalent of wavelength-division multiplexing, our technique performs the equivalent of code-division multiplexing. Design of a spread-spectrum encoder A key property of a SSE is that it should spread the direction of incoming rays as little as possible. To ensure this, we must first identify where such spreading comes from. In the case of a grating, it comes from lateral features in the grating structure. A SSE, therefore, should be essentially devoid of lateral features and as translationally invariant as possible. On the other hand, to impart spectral codes, it must produce wavelength-dependent time delays. An example of a SSE that satisfies these conditions is a low-finesse Fabry–Perot etalon (FPE), as illustrated in the inset of Fig. 1 . This is translationally invariant and thus does not alter ray directions. Moreover, different wavelengths travelling through the etalon experience different, multiple time delays owing to multiple reflections. These time delays also depend on ray direction, providing the possibility of angle–wavelength encoding. It is important to note that losses through such a device are in the axial (backward) direction only, as opposed to lateral directions. Hence, there is no slit effect as in the case of a grating, meaning that the full spectrum can be utilized for encoding, and losses can be kept to a minimum independent of pixel number. This advantage is akin to the Jacquinot [26] advantage in interferometric spectroscopy (also called the étendue advantage). 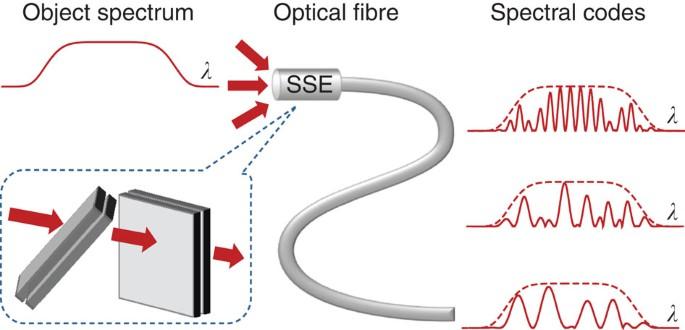Figure 1: Schematic of method. A self-luminous object with an extended spatial distribution produces light with a broad spectrum. Different spatial portions (pixels) of this object are incident on the entrance of an optical fibre from different directions. A spread-spectrum encoder (SSE) imparts a unique spectral code to each light direction in a power efficient manner. The resulting total spectrum at the output of the fibre is detected by a spectrograph, and image reconstruction is performed by numerical decoding. An example of a SSE is shown in the inset, consisting of two low-finesse Fabry–Perot etalons of different free spectral ranges, tilted perpendicular to each other to encode light directions in 2D. Figure 1: Schematic of method. A self-luminous object with an extended spatial distribution produces light with a broad spectrum. Different spatial portions (pixels) of this object are incident on the entrance of an optical fibre from different directions. A spread-spectrum encoder (SSE) imparts a unique spectral code to each light direction in a power efficient manner. The resulting total spectrum at the output of the fibre is detected by a spectrograph, and image reconstruction is performed by numerical decoding. An example of a SSE is shown in the inset, consisting of two low-finesse Fabry–Perot etalons of different free spectral ranges, tilted perpendicular to each other to encode light directions in 2D. Full size image A more detailed schematic of our setup is shown in Fig. 2 and described in Methods. To simulate an arbitrary angular distribution of self-luminous sources, we made use of a spatial light modulator (SLM) and a lens. The SLM was trans-illuminated by white light from a lamp and the lens’s only purpose was to convert spatial coordinates at the SLM to angular coordinates at the SSE entrance. The SSE here consisted of two FPEs in tandem, each tilted off axis so as to eliminate angular encoding degeneracies about the main optical axis (note: such tilting still preserves translational invariance). In this manner, each 2D ray direction within an angle spanning about 160 mrad, corresponding to our field of view, was encoded into a unique spectral pattern, which was then launched into a multimode fibre of larger numerical aperture. The light spectrum at the proximal end of the fibre was then measured with a spectrograph and sent to a computer for interpretation. 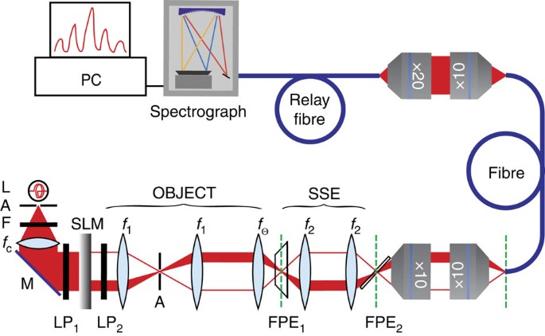Figure 2: Experimental setup for demonstration of spread-spectrum encoding. White light from a lamp is collimated with the use of a 1 mm aperture (A) and collimating lens (fc=100 mm). The light is directed through a transmission spatial light modulator (SLM). Crossed linear polarizers (LP1and LP2) ensure that the SLM provides amplitude modulation. A short-pass filter (F) is inserted to block wavelengths longer than 740 nm where the SLM contrast becomes degraded. A unit magnification relay (f1=100 mm) enables the insertion of a second 1 mm aperture (A) to remove spurious high-order diffracted light from the SLM. Lens (fθ=25 mm) has a key role in converting SLM pixel positions into ray directions. The spread-spectrum encoder (SSE) comprises two orthogonally tilted low-finesse Fabry–Perot etalons (FPE1and FPE2), separated by a unit magnification relay (f2=25 mm). The light exiting the SSE is relayed (unit magnification, 0.25NA objectives) to the entrance of a bare optical fibre of core diameter 200 μm. A secondary relay fibre with smaller core size (100 μm) serves to improve the spectral resolution of our spectrograph. The spectrum is recorded with a camera and sent to a computer (PC). The vertical dashed lines correspond to optical planes separated by unit magnification relays whose only purpose is to provide physical space to accommodate optical mounts. Figure 2: Experimental setup for demonstration of spread-spectrum encoding. White light from a lamp is collimated with the use of a 1 mm aperture (A) and collimating lens ( f c =100 mm). The light is directed through a transmission spatial light modulator (SLM). Crossed linear polarizers (LP 1 and LP 2 ) ensure that the SLM provides amplitude modulation. A short-pass filter (F) is inserted to block wavelengths longer than 740 nm where the SLM contrast becomes degraded. A unit magnification relay ( f 1 =100 mm) enables the insertion of a second 1 mm aperture (A) to remove spurious high-order diffracted light from the SLM. Lens ( f θ =25 mm) has a key role in converting SLM pixel positions into ray directions. The spread-spectrum encoder (SSE) comprises two orthogonally tilted low-finesse Fabry–Perot etalons (FPE 1 and FPE 2 ), separated by a unit magnification relay ( f 2 =25 mm). The light exiting the SSE is relayed (unit magnification, 0.25NA objectives) to the entrance of a bare optical fibre of core diameter 200 μm. A secondary relay fibre with smaller core size (100 μm) serves to improve the spectral resolution of our spectrograph. The spectrum is recorded with a camera and sent to a computer (PC). The vertical dashed lines correspond to optical planes separated by unit magnification relays whose only purpose is to provide physical space to accommodate optical mounts. Full size image Image retrieval In our lensless configuration, the optical angular resolution defined by the fibre core diameter was ~3 mrad, which was better (smaller) than the minimum angular pixel size (12 mrad) used to encode our objects. Moreover, these minimum object pixel sizes were large enough to be spatially incoherent, meaning that the spectral signals produced by the pixels could be considered as independent of one another, thus reducing SSE to a linear system. Specifically, for M input pixel elements (ray directions A m ) and N output spectral detection elements ( B n ), the SSE process can be written in a matrix form as B= M A, where each column in M corresponds to the spectral code for its associated object pixel. These spectral codes must be measured in advance before any imaging experiment; however, once measured, they are insensitive to fibre motion or bending. Once M is defined, then imaging can be performed. An arbitrary distribution of self-luminous sources (object pixels) leads to a superposition of spectral codes weighted according to their respective pixel intensities. A retrieval of this distribution (A) from a measurement of the total output spectrum (B), is then formally given by A= M + B, where M + is the pseudo-inverse of M (see Methods). While the high throughput of a SSE facilitates the efficient transmission of object brightness, this alone is not sufficient to guarantee that image retrieval will be reliable. As we will see below, the reliability and immunity to noise of image retrieval critically depends on the condition of M . For example, representative spectral codes and singular values of M obtained with our SSE are illustrated in Supplementary Fig. 1 . Ideally, the singular values should be as evenly distributed as possible, indicating highly orthogonal spectral codes. In our case, condition numbers of M were on the order of a few hundred, suggesting that our SSEs were not ideal and could be significantly improved in future designs. Nevertheless, despite these high condition numbers, we were able to retrieve 2D images up to 49 pixels in size (see Figs 3 and 4 , and Supplementary Fig. 2 ), with weak pixel brightnesses roughly corresponding to that of a dimly lit room. 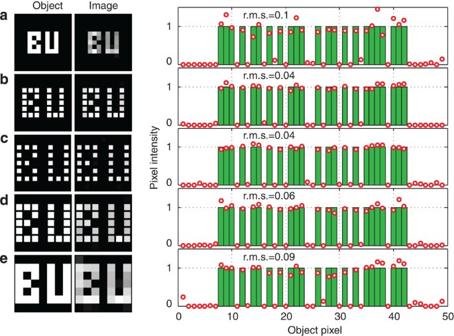Figure 3: Influence of pixel size and sparcity on spread-spectrum encoder (SSE) imaging. Spatially incoherent, white light objects in the shape of ‘BU’, consisting of 49 pixels (7 × 7), are sent through an SSE and launched into a fibre (see Methods). The reconstructed images and pixel values, along with associated r.m.s. errors, are displayed for different pixel layouts. In rows (a)–(c), the pixel sizes (powers) are the same, but their separation is increased, leading to better reconstruction (lower r.m.s. error). In rows (d) and (e), the pixel separations are the same, but their size is increased until the pixels are juxtaposed. The corresponding increase in pixel power is counterbalanced by a decrease in the contrast of associated spectral codes (due to increased angular diversity per pixel), leading to a net decrease in reconstruction quality (higher r.m.s.). The reconstructions were verified to be stable and insensitive to fibre movement or bending (seeSupplementary Fig. 3). Figure 3: Influence of pixel size and sparcity on spread-spectrum encoder (SSE) imaging. Spatially incoherent, white light objects in the shape of ‘BU’, consisting of 49 pixels (7 × 7), are sent through an SSE and launched into a fibre (see Methods). The reconstructed images and pixel values, along with associated r.m.s. errors, are displayed for different pixel layouts. In rows ( a )–( c ), the pixel sizes (powers) are the same, but their separation is increased, leading to better reconstruction (lower r.m.s. error). In rows ( d ) and ( e ), the pixel separations are the same, but their size is increased until the pixels are juxtaposed. The corresponding increase in pixel power is counterbalanced by a decrease in the contrast of associated spectral codes (due to increased angular diversity per pixel), leading to a net decrease in reconstruction quality (higher r.m.s.). The reconstructions were verified to be stable and insensitive to fibre movement or bending (see Supplementary Fig. 3 ). 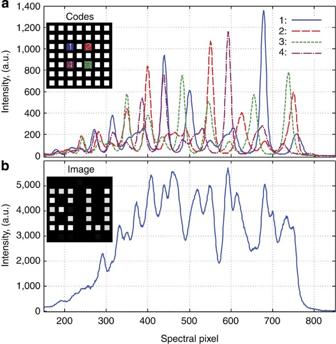Figure 4: Examples of spectral codes and detected spectrum. Spectral codes and output spectrum associated withFig. 2c. (a) Representative spectral codes (columns ofM) for four object pixels near centre (highlighted by different colours in the inset). (b) The total output spectrum (B) resulting from the weighted sum of spectra from all object pixels, here in the shape of ‘BU’ shown in the inset. One spectral pixel spans a wavelength of ~0.5 nm, leading to a full object bandwidth of ~300 nm. The spectral pixel marked 500 corresponds to 565 nm. Full size image Figure 4: Examples of spectral codes and detected spectrum. Spectral codes and output spectrum associated with Fig. 2c . ( a ) Representative spectral codes (columns of M ) for four object pixels near centre (highlighted by different colours in the inset). ( b ) The total output spectrum (B) resulting from the weighted sum of spectra from all object pixels, here in the shape of ‘BU’ shown in the inset. One spectral pixel spans a wavelength of ~0.5 nm, leading to a full object bandwidth of ~300 nm. The spectral pixel marked 500 corresponds to 565 nm. Full size image Number of resolvable pixels To evaluate the maximum number of resolvable object pixels that can be encoded by our SSE, we consider the idealized case where shot noise is the only noise source and begin by estimating the signal-to-noise ratio (SNR) for the image retrieval of a single pixel. We define W to be the total power that would be detected if no SSE were present in the system and all object pixels were full on throughout the entire field of view. We further define η to be the average transmissivity of the SSE (dependent on throughput), and γ to be a measure of the information content in the spectral codes defined by the coding matrix M (largely independent of throughput). This last parameter is difficult to quantify as it depends on the quality of the spectral codes, and thereby on the number of object pixels M enclosed in the field of view. Clearly, if the spectral codes are completely redundant ( γ =0), then no image information can be transmitted. A lower limit to γ can be roughly estimated by the inverse condition number of the coding matrix M (ref. 27 ). However, this lower limit can be significantly increased by applying dimensional reduction to M (that is, applying a minimum threshold to the singular values of M upon pseudo-inversion) or by applying priors during image reconstruction, such as a positivity constraint. In our case, with typical separations and sizes of M =49 object pixels and with the application of a positivity constraint, we attain values of γ of the order of 0.01 (though often a bit smaller). This is far short of the maximum value γ =1, which could be attained with ideal codes, and is an indication that there remains considerable room for improvement in the design of better SSEs. Continuing with our calculation, if the field of view is subdivided into M object pixels, then the detected energy per object pixel after passing through the SSE is ηWT / M , where T is the measurement time. In accord with the principle of spread-spectrum encoding, this energy is distributed in a roughly uniform manner over N detector (spectrograph) pixels, meaning that the average energy per detector pixel is ηWT / MN , and the corresponding r.m.s. noise per detector pixel is , where we assume that W is measured in units of photoelectrons per second and we neglect detector noise. But not all this average energy is useful. The energy per detection pixel that actually contains image information is γηWT / MN . We thus have a measure of signal and noise at the spectrograph. To calculate the signal and noise after image retrieval, we make the assumption that all the detected signals are correlated and thus contribute to the retrieved image signal in a coherent way (that is, scaling with N ), whereas all the detected noises are uncorrelated and contribute to the retrieved image noise in an incoherent way (that is, scaling with ). The SNR of the retrieved image per object pixel, assuming N > M , is thus where SNR B is the SNR associated with the detected spectrum B per object pixel (the first relation is in accord with ref. 27 ). This expression warrants scrutiny. First, let us examine how SNR A depends on M . As M increases, the power per object pixel W / M decreases, which is obviously detrimental to SNR A . On the other hand, as M decreases, provided the field of view remains fixed, the object pixels become larger in size, that is, they spread over larger solid angles. This increase in angular diversity per pixel generally leads to a decrease in the contrast γ of the spectral codes associated with each pixel. That is, both large and small M s are ultimately detrimental to SNR A . At first glance, it might appear that SNR A does not depend on N , until we note that γ depends on the contrast of the spectral codes upon detection. If N is large and the spectral codes are oversampled upon detection, then N has no effect on SNR A . On the other hand, if N is so small that the spectral codes are undersampled, then γ becomes reduced and accordingly, so does SNR A . In our case, η ~0.06 (corresponding to ~0.25 per dimension), ηW ~10 8 photoelectrons per second and T ≈1 s. For a desired SNR A of, say, 10, we obtain M roughly of the order of 100. This is an order of magnitude estimate, roughly in accord with our results. In summary, we have demonstrated a technique to perform imaging of self-luminous objects through a single optical fibre. The technique is based on encoding spatial information into spectral information that is immune to fibre motion or bending. A key novelty of our technique is that encoding is performed over the full spectral bandwidth of the system, meaning that high throughput is maintained independent of the number of resolvable image pixels (as opposed to wavelength-division encoding), facilitating the imaging of self-luminous objects. Encoding is performed by passive optical elements. In our demonstration, we made use of low-finesse FPEs, which exhibit no lateral structure and impart well-defined quasi-sinusoidal spectral codes whose periods depend on illumination direction. Alternatively, SSEs could impart much more complicated codes that are essentially random in structure, as obtained, for example, from a large number of stacked thin films of random thicknesses or refractive indices. SSE techniques based on pseudo-random codes are akin to asynchronous code-division multiplexing techniques in wireless communication. For our applications, these would render our image retrieval more immune to wavelength fading or colour variations in our object spectrum. It should be noted that spatio-spectral encoding based on randomly scattering media has already been demonstrated [23] , [24] ; however, in these cases, the scattering was roughly isotropic rather than 1D, which led to severe beam spreading and ultimately limited throughput. In principle, SSEs can be miniaturized and integrated within the optical fibre itself using photonic crystal or metamaterials techniques, or techniques similar to the imprinting of fibre Bragg gratings. Such integrated encoders should exhibit structure almost exclusively in the axial direction, though some weak lateral structure may be required to break lateral degeneracies and enable 2D angular encoding (leading to slight loss of contrast in the spectral codes). Yet, an alternative strategy to achieve 2D encoding is to perform 1D encoding with a SSE, and combine this with a physical translation or rotation of the optical fibre itself to achieve 2D imaging (similar to that in refs 18 , 22 ). This last alternative has the advantage that it can provide higher 2D image resolution, but has the disadvantage that it requires moving parts. While our demonstration here has been limited to proof of concept, we anticipate that applications of our technique include fluorescence or chemiluminescence micro-endoscopy deep within tissue. The narrower bandwidths associated with such imaging would require finer structures in our spectral codes and concomitantly higher spectral resolution in our spectrograph. Nevertheless, in principle, even highly structured encoding can be obtained, without loss of throughput and in an ultra-miniaturized geometry, leading to the attractive possibility of a micro-endoscopy device that causes minimal surgical damage. Alternatively, our technique could be used for ultra-miniaturized imaging of self-luminous or white light illuminated scenes for remote sensing. Optical layout The principle of our layout is shown in Fig. 1 and described in more detail in Fig. 2 . An incoherent (for example, self-luminous) object was simulated by sending collimated white light from a lamp through an intensity transmission spatial light modulator (Holoeye LC2002) with computer-controllable binary pixels. A lens ( f θ ) converted pixel positions into ray directions, which were then sent through the SSE and directed into an optical fibre (200 μm diameter, 0.39NA). The spectrum at the proximal end of the fibre was recorded with a spectrograph (Horiba CP140-103) featuring a spectral resolution of 2.5 nm as limited by the core diameter of a secondary relay fibre. SSE construction Our SSEs were made of two low-finesse FPEs tilted ~45° relative to the optical axis in orthogonal directions relative to each other. The FPEs were made by evaporating thin layers of silver of thickness typically 17 nm onto standard microscope coverslips, manually pressing these together to obtain air gaps of several microns and glueing with optical cement near the edges of the coverslips. Ideally the FPEs encoding orthogonal direction should exhibit very disparate free spectral ranges, however, this was difficult to achieve in our case. The finesse of FPE 1 was ~5, measured at 670 nm, with free spectral range of ~26 THz, indicating that the air gap was ~6 μm. The finesse of FPE 2 was ~3 at 670 nm, with free spectral range 19 THz and air gap ~8 μm. Calibration and image retrieval To determine the SSE matrix M before imaging, we cycled through each object pixel one by one and recorded the associated spectra (columns of M ). Recordings were averaged over 20 measurements with 800 ms spectrograph exposure times. Actual imaging was performed with single spectrograph recordings of B with 800 ms exposure times. Corresponding image pixels A m were reconstructed by least-squares fitting with a non-negativity prior, given by min A || M A−B|| 2 , where A m ≥0 ∀ m , as provided by the Matlab function lsqnonneg. We note that a baseline background spectrum obtained when all SLM pixels are off was systematically subtracted from all the spectral measurements to correct for the limited on/off contrast (about 100:1) of our SLM. How to cite this article : Barankov, R. and Mertz, J. High-throughput imaging of self-luminous objects through a single optical fibre. Nat. Commun. 5:5581 doi: 10.1038/ncomms6581 (2014).